Self-assembled two-dimensional nanofluidic proton channels with high thermal stability Exfoliated two-dimensional (2D) sheets can readily stack to form flexible, free-standing films with lamellar microstructure. The interlayer spaces in such lamellar films form a percolated network of molecularly sized, 2D nanochannels that could be used to regulate molecular transport. Here we report self-assembled clay-based 2D nanofluidic channels with surface charge-governed proton conductivity. Proton conductivity of these 2D channels exceeds that of acid solution for concentrations up to 0.1 M, and remains stable as the reservoir concentration is varied by orders of magnitude. Proton transport occurs through a Grotthuss mechanism, with activation energy and mobility of 0.19 eV and 1.2 × 10 −3 cm 2 V −1 s −1 , respectively. Vermiculite nanochannels exhibit extraordinary thermal stability, maintaining their proton conduction functions even after annealing at 500 °C in air. The ease of constructing massive arrays of stable 2D nanochannels without lithography should prove useful to the study of confined ionic transport, and will enable new ionic device designs. Exfoliation of layered materials in solution leads to dispersed single or few atomic/molecular layers that can be readily reassembled into paper-like films by filtration or casting [1] , [2] , [3] , [4] , [5] . The resulting films usually have a lamellar microstructure due to stacking of the high aspect ratio two-dimensional (2D) sheets. Such lamellar thin films, including those made of graphene-based sheets, have been extensively studied unveiling interesting mechanical, optoelectronic and electrochemical properties [6] , [7] , [8] . These high aspect ratio 2D sheets, regardless of material composition, have a unique advantage over other morphologies in that they are the only shape that can stack to yield continuous interstitial space, which is both percolated throughout the material and highly uniform in size and orientation. This offers unprecedented opportunity to construct nanofluidic channels to study molecular transport [9] , [10] , [11] , [12] . The width of such lamellar channels is comparable to the apparent thickness of the 2D sheets, and typically can be adjusted from around half a nanometre to several nanometres. This lengthscale is similar to the size of solvated ions as well as the Debye length of electrolytes at up to physiological concentrations. Many works have used similarly sized nanofluidic channels, fabricated by lithography or using a sacrificial template, to demonstrate that ions behave very differently in confined environments than they do in bulk [13] , [14] , [15] , [16] , [17] . For example, when the channel dimension becomes comparable to Debye length, ions carrying the opposite charge to the channel wall become enriched, and ions carrying the same charge as the channel wall are excluded. At this unipolar transport stage, ion concentration is determined by the surface charge on the channel wall rather than the bulk concentration, and the increased carrier concentration leads to enhanced ionic conductivity. Although it has been challenging to fabricate channels at this dimension, we have found that they can be rapidly generated in bulk scale and over macroscopic areas by restacking 2D sheets. In an earlier work, we discovered that the spaces between stacked graphene oxide sheets can indeed function as cation-selective nanofluidic channels for electrolytes [12] . Higher-than-bulk ionic conductivity, governed by the surface charge of the channel walls, was observed. High ionic conductivity in graphene and graphene oxide-based multilayer thin films has also been confirmed by others [18] , [19] . However, graphene oxide is thermally unstable [20] , [21] and can start to deoxygenate and lose its lamellar ordering before 200 °C. This greatly limits the use of graphene oxide-based lamellar membranes. Here we report a lamellar membrane constructed from exfoliated layers of a clay mineral, which exhibits high proton conductivity and extraordinary thermal stability. Clay minerals are naturally occurring phyllosilicates that can be found in sedimentary rocks and hydrothermal deposits, and have found widespread applications from the beginning of human civilization [22] , [23] . Compared with graphene oxide and other 2D materials, clay layers have significant advantages for constructing lamellar membranes for regulating molecular transport: (1) the starting material is much more readily available. (2) Clay layers can be exfoliated in water via ionic exchange, which is much more benign than chemical exfoliation of graphene and other 2D materials. (3) Clay layers have extraordinary chemical and thermal stability, and can withstand heating at elevated temperature over extended period of time without losing the lamellar ordering. (4) The structural diversity in the family of natural and synthetic clay minerals makes it possible to design 2D nanofluidic channels with desirable sign of charge and charge density. In this work, we select vermiculite as our model clay system to construct 2D nanofluidic channels. Synthesis and characterization of vermiculite nanochannels Vermiculite is a layered magnesium aluminosilicate compound with each layer composed of one Mg-based octahedral sheet sandwiched between two tetrahedral silicate sheets ( Fig. 1a ) [23] . Substitutional Al 3+ impurities in the tetrahedral sheets give rise to the negative charges on the layers, which are balanced by cations between the layers. Vermiculite crystals can be partially exfoliated by thermal shock, which rapidly vapourizes interlayer water and expands the crystals into an accordion-like structure ( Fig. 1b ). The flakes can then be swollen by several steps of ionic exchange to eventually replace the interlayer cations with Li + , which has a larger hydration diameter [24] . Finally, a hydrogen peroxide treatment is applied so that oxygen evolution from its decomposition helps to further exfoliate the vermiculite layers [25] . This chemical exfoliation processing yields a light brown colloidal suspension of vermiculite layers ( Fig. 2c ). The dispersion (1.5 mg ml −1 ) exhibits strong optical birefringence when seen through crossed polarizers ( Fig. 1d ), indicating nematic liquid crystalline ordering due to high aspect ratio of the dispersed layers [26] . The lateral dimension of the layers are from a few microns to tens of microns based on scanning electron microscopy (SEM) ( Fig. 1e ). 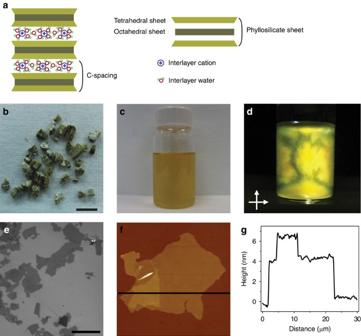Figure 1: Exfoliation of vermiculite crystals and resulting dispersions of few-layer flakes. (a) Structural model of vermiculite layers. (b) Thermally expanded vermiculite crystals (scale bar, 5 mm), which can be exfoliated by ion exchange to form (c) a single to few-layer dispersion in water. (d) The dispersion exhibits strong birefringence when viewed through crossed polarizers, suggesting nematic ordering originating from the high aspect ratios of the flakes. (e) SEM (scale bar, 50 μm). (f) Atomic force microscopy (AFM) image and (g) corresponding AFM height profile of exfoliated flakes shows that they are few-layer stacks with lateral dimensions of tens of microns. Figure 1f shows the atomic force microscopy image of a typical exfoliated vermiculite flake. The height profile ( Fig. 1g ) shows that the thinnest part of the flake is around 3 nm, indicating a bilayer [27] . The exfoliated vermiculite layers can be readily reassembled by vacuum filtration to form a light brown, paper-like flexible thin film ( Fig. 2a ) with lamellar microstructure as shown in the cross-sectional SEM image ( Fig. 2b ). The thickness of such vermiculite papers is determined by the concentration and volume of the colloidal dispersion used for filtration. Figure 1: Exfoliation of vermiculite crystals and resulting dispersions of few-layer flakes. ( a ) Structural model of vermiculite layers. ( b ) Thermally expanded vermiculite crystals (scale bar, 5 mm), which can be exfoliated by ion exchange to form ( c ) a single to few-layer dispersion in water. ( d ) The dispersion exhibits strong birefringence when viewed through crossed polarizers, suggesting nematic ordering originating from the high aspect ratios of the flakes. ( e ) SEM (scale bar, 50 μm). ( f ) Atomic force microscopy (AFM) image and ( g ) corresponding AFM height profile of exfoliated flakes shows that they are few-layer stacks with lateral dimensions of tens of microns. 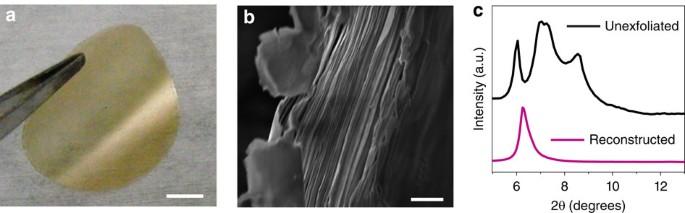Figure 2: Free-standing lamellar vermiculite membrane constructed from exfoliated flakes. (a) A flexible free-standing vermiculite membrane obtained by vacuum filtration (scale bar, 1 cm). The lamellar microstructure is clearly shown in (b) the cross-sectional SEM (scale bar, 1 μm). (c) XRD patterns of unexfoliated vermiculite crystals and the reconstructed vermiculite membranes. Full size image Figure 2: Free-standing lamellar vermiculite membrane constructed from exfoliated flakes. ( a ) A flexible free-standing vermiculite membrane obtained by vacuum filtration (scale bar, 1 cm). The lamellar microstructure is clearly shown in ( b ) the cross-sectional SEM (scale bar, 1 μm). ( c ) XRD patterns of unexfoliated vermiculite crystals and the reconstructed vermiculite membranes. Full size image While the starting vermiculite particles and the reassembled membrane both have lamellar structure, X-ray diffraction (XRD) studies revealed that they differ significantly in interlayer spacing. Vermiculite can have multiple interlayer spacing values owing to the presence of different interlayer cations, different degrees of hydration of the same interlayer cation or interstratified structures, which leads to more complex XRD patterns [28] . As shown in Fig. 2c , the XRD pattern of the thermally expanded vermiculite particles used in this work has four peaks in the 2 θ range of 5–15°. The peaks centred at 7.3° ( d 001 =12.1 Å) and 6.1° ( d 001 =14.5 Å) correspond to the {001} d -spacing of Mg-vermiculite with one and two hydration layers, respectively. The peak at 8.6° ( d 001 =10.3 Å) is attributed to the {001} diffraction of K-vermiculite and the peak at 7.1° ( d 001 =12.4 Å) is attributed to an interstratified layer spacing in between two forms of vermiculite. After ionic exchange and reassembly of the exfoliated layers, the XRD pattern of the vermiculite membrane shows a single distinct peak at 2 θ =6.2°. The corresponding d 001 spacing 14.1 Å is in agreement with that of lithium-intercalated vermiculite, indicating that the original interlayer cations (Mg 2+ , K + ) have been successfully exchanged. The exfoliation-reassembly process effectively creates a more uniform lamellar structure with well-defined interlayer spacing. The highly ordered lamellar structure of the vermiculite films makes it possible to correlate their degree of hydration to interlayer spacing, which can be conveniently measured by XRD. Over the course of exfoliation and filtration, vermiculite sheets become amply hydrated. The prominent {001} peak of the reconstructed membrane at around 6.2° corresponds to the interlayer spacing of fully hydrated vermiculite with two intercalated water monolayers [28] . Its not surprising that the reconstructed lamellar films are well hydrated, since the layers are exfoliated and reassembled in water. If the vermiculite membranes were less hydrated, larger angle peaks at 7°<2 θ <10° would appear. The absence of such peaks in the XRD pattern ( Fig. 2c ) suggests that the vermiculite nanochannels are fully hydrated. Therefore, the volume of the interlayer space is considered to be fully wetted by water. Surface charge-governed proton transport The proton conductivity through the nanofluidic channels in vermiculite films can be conveniently measured as illustrated in Fig. 3a . To make two terminal d.c. measurements, a rectangular vermiculite membrane was embedded in a polydimethylsiloxane (PDMS) elastomer with its two ends exposed to acid solutions. The photograph in Fig. 3b shows a complete device. Three representative current−voltage ( I − V ) curves recorded at different HCl concentrations are shown in Fig. 3c . Conductance is then calculated based on the slope of the I − V curves. From conductance, ionic conductivity is calculated based on the effective dimensions of the 2D channels (see Methods). 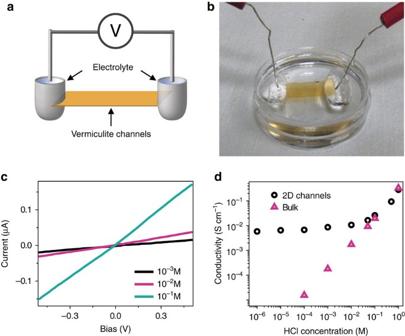Figure 3: Surface charge-governed proton transport through vermiculite channels. (a) Schematic illustration and (b) photo of the vermiculite nanofluidic device. (c) RepresentativeI–Vcurves through the 2D channels. (d) Ionic conductivity as a function of electrolyte concentration. The deviation from bulk solution at low proton concentration is characteristic of surface charge-governed transport. Figure 3d shows the pH-dependent ionic conductivity through the vermiculite nanochannels in comparison with that of the bulk HCl solution. The conductivity of bulk HCl solution is largely proportional to concentration ( Fig. 3d , red triangles). At high concentration, conductivity values of vermiculite channels are similar to that of bulk; however, conductivity through the nanochannels deviates from the bulk behavior for HCl concentration below 0.1 M ( Fig. 3d , black circles). Below 0.01 M, channel conductivity is rather constant and independent of bulk acid concentration, which is a signature of surface charge-governed transport. In this regime of acid concentration, the Debye length near the negatively charged vermiculite layer is greater than the interlayer spacing. Therefore, cations are the dominant charge carrier, and their concentration inside the channels is determined by the surface charge density rather than bulk electrolyte concentration. The successful observation of surface charge-governed transport also indicates good sealing of the vermiculite paper by PDMS, as short circuit ionic conductance due to leakage would likely exhibit bulk behaviour. Figure 3d shows that the fully hydrated vermiculite channels exhibit high proton conductivity of 6.0 × 10 −3 S cm −1 at near-neutral aqueous solution, which gradually increases to 2.6 × 10 −2 S cm −1 as pH value decreases to 1. A surface charge-governed transport mechanism explains the observation of greater-than-bulk proton conductivity through the 2D channels that varies less than fivefold as proton concentration changes over five orders of magnitude. Figure 3: Surface charge-governed proton transport through vermiculite channels. ( a ) Schematic illustration and ( b ) photo of the vermiculite nanofluidic device. ( c ) Representative I–V curves through the 2D channels. ( d ) Ionic conductivity as a function of electrolyte concentration. The deviation from bulk solution at low proton concentration is characteristic of surface charge-governed transport. Full size image Effects of isotope and temperature on proton transport To study the temperature effect on nanofluidic ionic current, a vermiculite membrane is embedded into a PDMS block along with a thermometer, and the PDMS block is heated in an oil bath, as shown schematically in Fig. 4a . The conductance of the vermiculite follows an Arrhenius-like behaviour, as shown in Fig. 4b , with activation energy of 0.19 eV. The low activation energy suggests that protons are transported through vermiculite nanochannels by a Grotthuss mechanism [29] , [30] , [31] . In this mechanism, charge is transported by the coordinated hopping of protons between water molecules in the nanochannels. This mechanism is consistent with the structural model of vermiculite, in which a continuous network of water molecules fills the galleries between layers ( Fig. 1a ). 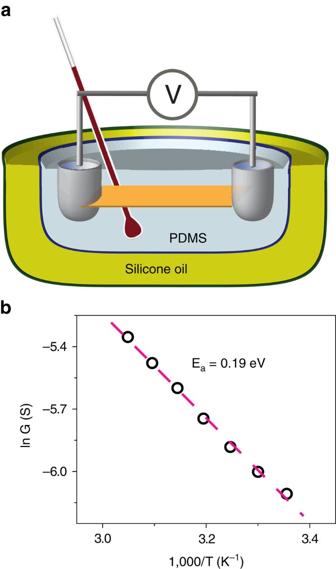Figure 4: Effect of temperature on proton transport. (a) Schematic illustration of experimental set-up for temperature-dependent conductance measurements. A vermiculite strip and a thermometer are embedded in PDMS, and heated via a silicone oil bath. (b) Arrhenius plot of proton conductance though the 2D channels. Figure 4: Effect of temperature on proton transport. ( a ) Schematic illustration of experimental set-up for temperature-dependent conductance measurements. A vermiculite strip and a thermometer are embedded in PDMS, and heated via a silicone oil bath. ( b ) Arrhenius plot of proton conductance though the 2D channels. Full size image To confirm protonic conductivity, we exchange H + with D + by soaking devices in deuterated electrolyte baths for 2 days. The conductance of the devices, initially measured in H 2 O, decreases by a factor of 1.6±0.1 after being soaked in D 2 O, and is largely restored after exchanging the electrolyte back to H 2 O. The isotope effect observed here is in line with the isotope effect values expected for Grotthuss transport ( ∼ 1.5) as opposed to vehicular transport (where the ideal isotope effect equals the viscosity ratio, ∼ 1.2) [32] , [33] . Surface charge density and proton mobility Surface charge density, σ S , is inferred from the ionic exchange capacity of vermiculite, which is a commonly used strategy for determining surface charge density for other proton conductors [34] . A vermiculite membrane ( ∼ 100 mg dry weight) is first oven dried until Fourier transform infrared spectroscopy indicates the complete removal of water. Then it is immersed in 2 ml of 1 mM HCl overnight, after which it exfoliates [35] . The H + in the solution exchanges with the Li + ions in the interlayer spaces, and the conductivity of the electrolyte drops owing to the conductivity difference between HCl (limiting conductance 425 Ω −1 ) and LiCl (limiting conductance 115 Ω −1 ) [36] . The change in solution conductivity of the supernatant is used to infer the amount of H + that had changed to Li + , and the presence of lithium in the dried supernatant is confirmed by X-ray photoelectron spectroscopy. The total surface area of the film can be calculated from its mass, density and interlayer spacing. From all of this, the surface charge density is calculated to be 1.4 mC m −2 and proton mobility 1.2 × 10 −3 cm 2 V −1 s −1 . For comparison, the mobility of vermiculite is comparable to what has been seen in the commercial proton conductor Nafion [34] , [37] . Alternatively, as shown in literature [16] , surface charge density could also be estimated from the graph of concentration versus conductivity (for example, Fig. 3d ) based on a set of simplified hypotheses ( Supplementary Fig. 1 , Supplementary Note 1 ). As the aligned 2D channels favours in-plane proton transport, further work is needed to reorient the channels to yield the high cross-plane conductivity needed for typical membrane applications. Thermal stability of vermiculite nanofluidics An advantage of using clay layers rather than organic materials or graphene-based materials to construct proton channels is their extraordinary thermal stability. Thermogravimetric analysis of the vermiculite membrane ( Fig. 5a ) shows that it initially experiences a rapid weight loss of about 4.8% on heating to 100 °C in air and another 1.2% by 200 °C. Next, it experiences a slow weight loss of an additional 5% and becomes stable after reaching 855 °C. XRD studies ( Fig. 5b ) revealed that annealing the membrane at 200 °C for a day does not affect its interlayer spacing, suggesting that the initial 6% weight loss observed in thermogravimetric analysis might be due to removal of physisorbed water. The interlayer spacing decreases from 14.1 to 9.8 Å after annealing at 500 °C due to removal of interlayer water molecules. However, the membrane can be readily rehydrated, expanding its interlayer spacing ( Fig. 5b ). After annealing at 900 °C, the membrane still maintains the lamellar structure, but became very brittle and hard to handle. 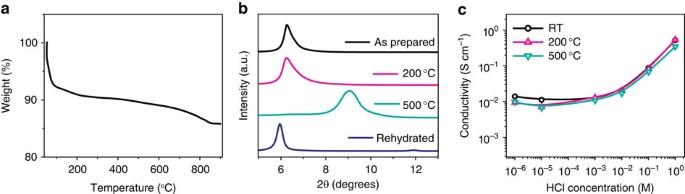Figure 5: Thermal stability of vermiculite-based proton channels. (a) Thermogravimetric analysis plot of a restacked vermiculite film. (b) XRD shows that the vermiculite film retains its interlayer spacing after heating at 200 °C. The spacing shrinks as the membrane dehydrates from heating for a day at 500 °C, but is restored on rehydration. (c) The proton conductivity of a vermiculite membrane is largely unaffected when dried at 200 °C or annealed at 500 °C for 1 day. Figure 5c compares proton conductivities through a vermiculite membrane at different pH values before and after thermal annealing in air for 1 day. The conductivity of vermiculite membrane does not exhibit significant change due to annealing at 200 °C, or even 500 °C. Figure 5: Thermal stability of vermiculite-based proton channels. ( a ) Thermogravimetric analysis plot of a restacked vermiculite film. ( b ) XRD shows that the vermiculite film retains its interlayer spacing after heating at 200 °C. The spacing shrinks as the membrane dehydrates from heating for a day at 500 °C, but is restored on rehydration. ( c ) The proton conductivity of a vermiculite membrane is largely unaffected when dried at 200 °C or annealed at 500 °C for 1 day. Full size image Thermally stable 2D proton channels can be readily constructed by the restacking of exfoliated vermiculite sheets. Surface charge-governed proton conductivity, exceeding that of bulk solution, is observed for pH values <1. Vermiculite channels show consistent conductance over orders of magnitude variations in proton concentration. Isotope and temperature effects suggest a proton transport mechanism based on hopping through the interlayer water molecules. Surface charge density on the vermiculite walls and proton mobility were determined to be around 1.4 mC m −2 and 1.2 × 10 −3 cm 2 V −1 s −1 , respectively. The vermiculite films have extraordinary thermal stability. They maintain their layered structures even after annealing in air at elevated temperatures, and can be readily rehydrated to restore ionic conductivity. These lamellar clay membranes are a model system to construct nanofluidic devices and materials. They can be assembled at unprecedentedly large scale with cheap materials and simple processing techniques, lowering the barrier of entry for studying confined ionic behaviours. This, in addition, establishes a readily accessible platform to accelerate discoveries in potential applications of nanofluidics such as sensing, catalysis and energy harvesting [38] , [39] , [40] . The work here also provides a new example of collective properties of bulk nanostructured materials, where new ionic transport behaviors emerge upon rational assembly of nanoscale building blocks. Chemicals Thermally expanded vermiculite crystals, sodium chloride, potassium chloride, lithium chloride, deuterium oxide and deuterochloric acid were purchased from Sigma Aldrich and used as received. Aqueous hydrogen peroxide (H 2 O 2 ) and hydrochloric acid were purchased from Avandor Performance Materials and used as received. Preparation of vermiculite membranes The thermally expanded vermiculite crystals were subjected to a two-step ion-exchange method. Fifty mg of vermiculite crystals soaked in a saturated sodium chloride (NaCl) solution were heated under reflux for 24 h, followed by vacuum filtration and repeated washing with deionized water and ethanol. The as-obtained product was again soaked in 2 M lithium chloride (LiCl) solution and was heated under reflux for an additional 24 h, followed by vacuum filtration and extensive washing with deionized water and ethanol. The product was then dispersed in water with the help of magnetic stirring and centrifuged at 6,000 r.p.m. for 10 min to obtain a jelly-like vermiculite slurry. Finally, the supernatant slurry was filtered through an anodic alumina membrane to obtain light yellow coloured flexible vermiculite films, which can be easily peeled off on drying. Characterization The thickness of the exfoliated vermiculite layers was determined by atomic force microscopy, XE-100, Park System. The thickness of the membranes was determined by profilometry (Dektak 150) or cross-sectional SEM The proton transportation measurements were carried out on a probe station equipped with a Keithley 2601A source meter inside a Faraday cage. XRD patterns were recorded using a Rigaku SmartLab diffractometer with Cu Kα radiation. Preparation of the nanofluidic devices To fabricate the membrane-based nanofluidic devices, membranes were cut into rectangular pieces and immersed into a blend of PDMS prepolymer and curing agent. After curing, two reservoirs were carved out in the PDMS device to expose the two ends of the membrane to the electrolyte solutions. More details about our device making process can be found in our previous article [12] . Conductivity measurement of the nanofluidic devices Two Ag/AgCl electrodes were inserted into both the source and drain reservoirs to measure proton current through the membranes. The representative I−V curves of the membrane-based nanofluidic devices were recorded at different HCl concentrations, ranging from 10 −6 M to 1 M. The conductivity was calculated based on the measured physical dimensions of the membranes and the interlayer spacing. XRD results suggest that the interlayer space is fully hydrated, and corresponds to about 34% of the total thickness of the thin film. Therefore, for the calculations of channel conductivity, the collective channel thickness of the films was taken as 34% of the membrane thickness determined by profilometry and confirmed by cross-sectional SEM. Measurement of surface charge density by ionic exchange The surface charge density of a dry vermiculite film was determined by an ionic exchange method. As-prepared vermiculite membranes were oven dried until the –OH band at 3,200–3,400 cm −1 is absent from their Fourier transform infrared spectroscopy spectrum, indicating the complete removal of water. Next 100 mg of dried membrane was soaked in 2 ml of 1 mM HCl overnight. The change in solution conductivity of the supernatant was used to infer the amount of H + that had been replaced by released interlayer Li + , which can be used to calculate surface charge density. The supernatant was cast onto a Si wafer and dried. The presence of LiCl was confirmed by X-ray photoelectron spectroscopy measurements. Effects of temperature and isotope on conductivity To study the temperature effects on ionic current, a nanofluidic device was made by implanting a thermometer into a PDMS block along with the vermiculite membrane. The ends of the membrane were exposed to 10 −4 M HCl solution through the carved reservoirs. The acid-soaked device was then immersed into an oil bath that was heated at a rate of 0.2 °C min −1 from room temperature to 80 °C. At regular intervals, the ionic conductance was recorded by measuring I–V curves, while the temperature was measured by the embedded thermometer. For isotope effect measurements, vermiculite nanofluidic devices were soaked alternately in H 2 O and D 2 O solvent for extended time ( ∼ 24 h), to ensure complete hydration. After conductance was measured at particular solvent, devices were dried at 75 °C in air for 24 h before switching solvents. Thermal stability of vermiculite nanochannels The vermiculite membranes were placed on glass slides and heated in a muffle furnace at 200 and 500 °C in air for a day. To avoid exfoliation and complete disintegration of the membrane in water [35] , rehydration was done by adding a small aliquot of water that was just enough to cover the glass-supported membrane. XRD pattern was then acquired on the water-covered membrane after soaking overnight. How to cite this article: Shao, J.-J. et al. Self-assembled two-dimensional nanofluidic proton channels with high thermal stability. Nat. Commun. 6:7602 doi: 10.1038/ncomms8602 (2015).